Wnt signalling underlies the evolution of new phenotypes and craniofacial variability in Lake Malawi cichlids Progress towards understanding adaptive radiations at the mechanistic level is still limited with regard to the proximate molecular factors that both promote and constrain evolution. Here we focus on the craniofacial skeleton and show that expanded Wnt/ β -catenin signalling early in ontogeny is associated with the evolution of phenotypic novelty and ecological opportunity in Lake Malawi cichlids. We demonstrate that the mode of action of this molecular change is to effectively lock into place an early larval phenotype, likely through accelerated rates of bone deposition. However, we demonstrate further that this change toward phenotypic novelty may in turn constrain evolutionary potential through the corresponding reduction in craniofacial plasticity at later stages of ontogeny. In all, our data implicate the Wnt pathway as an important mediator of craniofacial form and offer new insights into how developmental systems can evolve to both promote and constrain evolutionary change. Adaptive radiations arise as a lineage evolves to fill newly available ecological niches, and can result in the production of both continuous and discontinuous phenotypic variation [1] . The efficiency by which this process occurs depends on numerous factors, including, but not limited to, the underlying genetic and developmental architectures of adaptive traits. Genetic architecture, sometimes referred to as the genotype–phenotype map, refers to how variation at the genetic level translates to phenotypic variation [2] . However, it is often not appreciated that the genotype–phenotype map interacts with environmental conditions over the course of development, and this interaction plays a major role in determining the patterns of variation that are exposed to selection through phenotypic plasticity [3] , [4] . Notably phenotypic plasticity is itself a trait that can evolve to suit conditions, with consistently variable environments favoring an increase in the magnitude of plasticity, and stable conditions favoring a reduction in plasticity due to its costs [4] , [5] . In accordance with this, models of adaptive divergence have predicted that increasing ecological specialization should result in a concomitant reduction in phenotypic plasticity [6] . Such models therefore predict a tradeoff between ecological specialization and phenotypic variability, and suggest that molecular changes that lead to the production of novel/extreme adaptations may come at the expense of an ability to respond to environmental changes. East-African cichlids are unquestionably one of the most successful adaptive radiations of any living organism, making them an ideal model in which to examine phenotypic evolution in the context of rapid diversification. Here we use cichlid fishes from Lake Malawi to examine the genetic and developmental basis for eco-morphological novelty and to assess whether such innovations have come at the expense of phenotypic variability/plasticity. Given its putative adaptive significance [7] , [8] , we focused on the preorbital region of the skull, which contains both the upper and lower jaws as well as the anterior skull ( Fig. 1 ). Further, variation in the length and profile of this region represents the major axis of phenotypic divergence among Lake Malawi cichlids [7] . Species on one end of this axis have long jaws, a shallow preorbital profile of the skull, and forage from the water column. Species on the opposite end possess short jaws, steeply rounded profiles, and forage from the benthos. Our experiments were intended to modulate trophic architecture through both feeding treatments (that is, ecologically relevant environmental perturbation) and the application of pharmacological compounds during craniofacial development (that is, molecular perturbation). We focus on Wnt signalling because of its known role in mediating vertebrate craniofacial development [9] and variation [10] , and putative role in distinguishing cichlid species with alternated jaw morphologies [11] . We demonstrate that expanded Wnt signalling is associated with the evolution of a novel skull morphology in Lake Malawi cichlids, possibly by promoting earlier and more robust ossification of the craniofacial skeleton. We show further that this divergent phenotype is better able to buffer against environmental change, an attribute that may underlie the ecological success of this group, but could also have a negative effect on its capacity for future evolutionary change. In all, our data provide empirical evidence of a potential tradeoff between the evolution of phenotypic novelty and evolutionary potential. 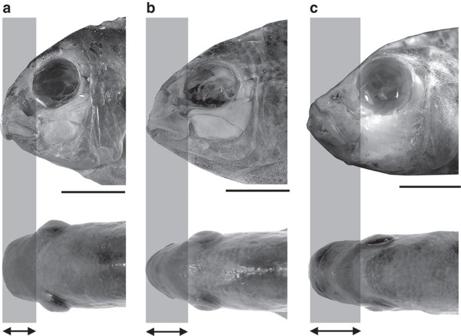Figure 1: Representative rock-dwelling cichlid species from Lake Malawi. The fish are shown in the lateral and dorsal views, and exhibit a range of variation with respect to the length of the preorbital region of the skull (shaded grey). From relatively short to relatively long: LF,Labeotropheus fuelleborni(a); TRC,Tropheopssp. ‘red cheek’ (b); MZ,Maylandia zebra(c), respectively. Lateral images are of dissected specimens that have had their eyes removed and skin deflected to reveal salient bones and muscles of the feeding apparatus. Scale bars, 1 cm. Figure 1: Representative rock-dwelling cichlid species from Lake Malawi. The fish are shown in the lateral and dorsal views, and exhibit a range of variation with respect to the length of the preorbital region of the skull (shaded grey). From relatively short to relatively long: LF, Labeotropheus fuelleborni ( a ); TRC, Tropheops sp. ‘red cheek’ ( b ); MZ, Maylandia zebra ( c ), respectively. Lateral images are of dissected specimens that have had their eyes removed and skin deflected to reveal salient bones and muscles of the feeding apparatus. Scale bars, 1 cm. Full size image Wnt signalling is active in the developing skull A recent genomic survey among Malawi cichlids revealed a synonymous polymorphism in β-catenin , a key member of the Wnt signalling pathway, that is nearly alternatively fixed between two species, Labeotropheus fuelleborni (LF) and Maylandia zebra (MZ) [11] . These species exhibit alternate jaw morphologies along the major axis of cichlid divergence, with LF possessing an extremely shortened jaw and steep craniofacial profile relative to other species of cichlids from the African rift lakes, while MZ possesses an intermediate jaw morphology. We therefore focused our experiments on these rock-dwelling species. Given the known roles for Wnt signalling in regulating bone development in general [12] and craniofacial development in particular [9] we sought to examine the role for this pathway in the development and evolution of the cichlid skull. We predicted that Wnt pathway members would be expressed within the preorbital region of the teleost skull during craniofacial development. To test this prediction in cichlids, we used whole-mount in situ hybridization (WISH) assays using both β-catenin , an intracellular signalling component of the canonical Wnt pathway, and lef1 , a downstream member of the Wnt pathway. β-catenin is broadly expressed in cichlid larva, with discrete expression observed within the pharyngeal arches, pectoral girdle (that is, cleithrum), pectoral fin pad, medial fin fold and caudal fin ( Supplementary Fig. 1 ). Discrete expression of both β-catenin and lef1 was also observed within the developing preorbital region of the skull, and was especially strong in LF. Wnt activity was detected just before (for example, st 17; Fig. 2 ) and during (for example, st 18; Fig. 2 ; Supplementary Fig. 2 ) preorbital outgrowth ( Fig. 2 , white outlined regions). We next set out to assess the degree to which craniofacial Wnt signalling in zebrafish matched that observed in cichlids. Here we used a transgenic Wnt reporter line, Tg ( 7xTCF-Xla.Siam:GFP ), to assess transcriptional activities controlled by Wnt/β-catenin signalling during craniofacial development. We note clear GFP expression in the developing preorbital region of the zebrafish head between 48–72 h post-fertilization ( Fig. 3 ). This pattern of expression is markedly similar to that observed in cichlids, and suggests an evolutionarily conserved role for Wnt signalling during craniofacial development across bony fishes. 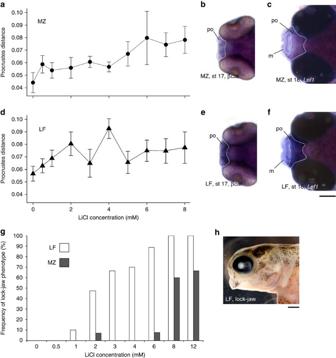Figure 2: The phenotypically derived species has higher endogenous levels of Wnt signalling during craniofacial development. (a) The phenotypically intermediate species, MZ, exhibits a gradual response to increasing concentrations of LiCl with respect to craniofacial shape (n=264, error bars are s.e.). This species also shows relatively low levels of Wnt signalling in the preorbital region of the skull at stage 17 (b) just before outgrowth of the preorbital (po) region of the skull, and stage 18 (c) just after outgrowth has commenced. (d) Alternatively, the phenotypically novel species, LF, exhibits a far more pronounced and erratic response to increasing concentrations of LiCl with respect to craniofacial shape (n=230, error bars indicate s.e.). LF also exhibits relatively higher levels of Wnt signalling in the preorbital region of the skull at stages 17 (e) and 18 (f). For both species, the response of craniofacial shape to LiCl treatment was measured as procrustes distance (PD) from the mean shape of MZ control fish (g). The phenotypically novel species, LF, also exhibits a far more pronounced response to low concentrations of LiCl with respect to the development of a lethal, lock-jaw, phenotype (h). In particular, approximately half of LF larvae develop locked jaws with 2 mM of LiCl, whereas 8 mM of LiCl is required to elicit a similar frequency of lock-jaw larvae in MZ. Collectively, these experiments suggest that LF larvae possess higher levels of Wnt signalling during craniofacial development compared to MZ. Scale bars, 200 μm. Figure 2: The phenotypically derived species has higher endogenous levels of Wnt signalling during craniofacial development. ( a ) The phenotypically intermediate species, MZ, exhibits a gradual response to increasing concentrations of LiCl with respect to craniofacial shape ( n =264, error bars are s.e.). This species also shows relatively low levels of Wnt signalling in the preorbital region of the skull at stage 17 ( b ) just before outgrowth of the preorbital (po) region of the skull, and stage 18 ( c ) just after outgrowth has commenced. ( d ) Alternatively, the phenotypically novel species, LF, exhibits a far more pronounced and erratic response to increasing concentrations of LiCl with respect to craniofacial shape ( n =230, error bars indicate s.e.). LF also exhibits relatively higher levels of Wnt signalling in the preorbital region of the skull at stages 17 ( e ) and 18 ( f ). For both species, the response of craniofacial shape to LiCl treatment was measured as procrustes distance (PD) from the mean shape of MZ control fish ( g ). The phenotypically novel species, LF, also exhibits a far more pronounced response to low concentrations of LiCl with respect to the development of a lethal, lock-jaw, phenotype ( h ). In particular, approximately half of LF larvae develop locked jaws with 2 mM of LiCl, whereas 8 mM of LiCl is required to elicit a similar frequency of lock-jaw larvae in MZ. Collectively, these experiments suggest that LF larvae possess higher levels of Wnt signalling during craniofacial development compared to MZ. Scale bars, 200 μm. 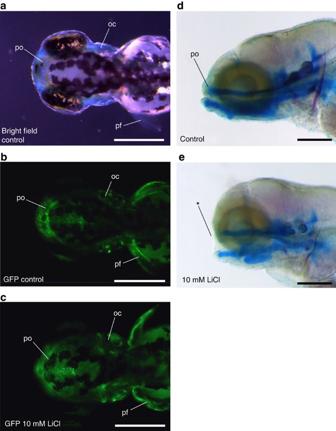Figure 3: Wnt signalling is associated with the development of the preorbital region of the zebrafish skull. (a,b) At 48 hours post fertilization (hpf) the Wnt report line,Tg(7xTCF-Xla.Siam:GFP), shows a clear and distinct output in Wnt signalling in the preorbital (po) domain of the zebrafish skull. (c)Tgzebrafish treated with LiCl exhibit a marked expansion of GFP expression in the po region of the skull, which suggests that LiCl treatment has a direct effect on Wnt signalling in this anatomical region. (d-e) Zebrafish treated with 10 mM of LiCl at 48hpf, show a marked reduction in preorbital outgrowth at 120 hpf. Asterisks in (e) indicates an apparent absence of the preorbital region of the skull. Scale bars, 200 μm. Full size image Figure 3: Wnt signalling is associated with the development of the preorbital region of the zebrafish skull. ( a , b ) At 48 hours post fertilization (hpf) the Wnt report line, Tg (7xTCF-Xla.Siam:GFP), shows a clear and distinct output in Wnt signalling in the preorbital (po) domain of the zebrafish skull. ( c ) Tg zebrafish treated with LiCl exhibit a marked expansion of GFP expression in the po region of the skull, which suggests that LiCl treatment has a direct effect on Wnt signalling in this anatomical region. ( d-e ) Zebrafish treated with 10 mM of LiCl at 48hpf, show a marked reduction in preorbital outgrowth at 120 hpf. Asterisks in ( e ) indicates an apparent absence of the preorbital region of the skull. Scale bars, 200 μm. Full size image An extreme phenotype exhibits higher levels of Wnt signalling The cichlid species LF has an extreme feeding apparatus relative to other African rift-lake cichlid species, characterized by a short and severely rounded craniofacial profile [7] . It is also one of the most cosmopolitan species within Lake Malawi, found at nearly every rocky outcrop, suggesting that its novel craniofacial architecture has facilitated its ecological success. Several lines of evidence suggest that this species also has endogenously higher levels of Wnt signalling during key stages of craniofacial development. First, the results of WISH analyses are consistent with LF having higher Wnt activity. Specifically, both β-catenin and lef1 are more robustly expressed in the preorbital region of the skull in LF relative to MZ (dotted outlines, Fig. 2 ). Consistent with these expression analyses, we find that in comparison to MZ, LF is far more sensitive to treatment with LiCl, a Wnt agonist that upregulates the pathway through inhibition of GSK3 (ref. 13 ). When treated with LiCl at stage 17, just before preorbital outgrowth, both LF and MZ exhibited a dose-dependent response in craniofacial shape, as measured by Procrustes distance (PD) at stage 23 (MANOVA, factor=concentration, F =10.1247 54,437 , P <0.001). However, we also document a significant dose by species effect (MANOVA; factor=species × concentration, F =4.1581 54,437 , P <0.001), with LF animals exhibiting a stronger dose-dependent response in craniofacial shape compared with MZ ( Fig. 2a,b ). In particular, craniofacial shape change (that is, PD from the mean MZ control configuration) due to LiCl treatment increased gradually in MZ ( Fig. 2a ), and only after animals were exposed to relatively high concentrations of LiCl (6–8 mM). LF animals, on the other hand, exhibited a far more acute and variable response ( Fig. 2b ) beginning with much lower levels of LiCl (that is, 2 mM). Notably, PD between control MZ and LF (0.015) was similar to that between control MZ and those treated with low doses of LiCl (0.015–0.02), and remained constant through an order of magnitude increase in LiCl exposure (0.5–4 mM). Over the same treatment range LF animals exhibited a strong and highly variable response in terms of craniofacial shape, with PD values ranging from 0.065 to 0.095. In both species, PD plateaued at ~0.075 with higher concentrations of LiCl (6–8 mM). Combined with the expression data, results from this LiCl experiment are consistent with the hypothesis that compared to MZ, LF has endogenously higher levels of Wnt signalling, making it far more sensitive to LiCl treatment. Further support for this hypothesis comes from the observation that treatment of cichlid larvae with higher doses of LiCl induced what we refer to as a ‘lock jaw’ phenotype, whereby the upper and lower jaws of the embryo became agape and immobile (animals died soon after developing this phenotype). The lock jaw phenotype is characterized by a steeply descending craniofacial profile, as well as more widespread developmental defects in the pharyngeal skeleton ( Supplementary Fig. 3 ). LF displayed a far more acute response to LiCl with respect to this phenotype ( Fig. 2c ). The lock jaw phenotype appeared at a high frequency in this species with nearly an order of magnitude less LiCl compared with MZ. Specifically, over half of the LF larvae treated with 2 mM of LiCl developed a lock jaw phenotype, whereas it took 8 mM LiCl before a similar proportion of MZ animals developed this phenotype. In all, data from expression analyses and LiCl treatment are consistent with the hypotheses that (1) Wnt signalling is involved in the development of the preorbital region of the skull in bony fishes, and (2) different levels of Wnt signalling underlie the development of species-specific skull shapes. Manipulation of Wnt signalling mimics natural jaw variation Developmentally, outgrowth of the preorbital region of the skull is initiated soon after hatching in Lake Malawi cichlids (stage 17, 5 days post fertilization(dpf)), and closely related species exhibit measurable differences in preorbital length by stage 23 (10 dpf, Fig. 4a–d ). To assess a role for Wnt signalling in mediating this process, we treated animals at stage 17 with both the Wnt agonist LiCl and the Wnt antagonist IWR-1 (ref. 12 ). Treatment of MZ, the species with an intermediate and putatively ancestral phenotype (and relatively low levels of Wnt), with LiCl resulted in a striking phenocopy of the derived condition. Specifically, MZ treated with LiCl at stage 17, just before the onset of preorbital expansion, exhibited a morphological phenotype with a severely rounded craniofacial profile similar to that of comparably staged LF larvae ( Fig. 4e,f ). To assess the degree to which the craniofacial skeleton responds to LiCl treatment is evolutionarily conserved, we repeated this experiment in comparably staged Wnt reporter zebrafish larvae using a similar concentration of LiCl (that is, 10 mM). We demonstrate that treatment with LiCl results in a marked expansion of Wnt signalling in the preorbital region of the skull ( Fig. 3c ). Furthermore, we show that treated zebrafish develop a severely rounded craniofacial profile ( Fig. 3e ), similar to that observed in treated cichlids, which suggests a high degree of conservation in the effects of elevated Wnt on preorbital development across fishes. 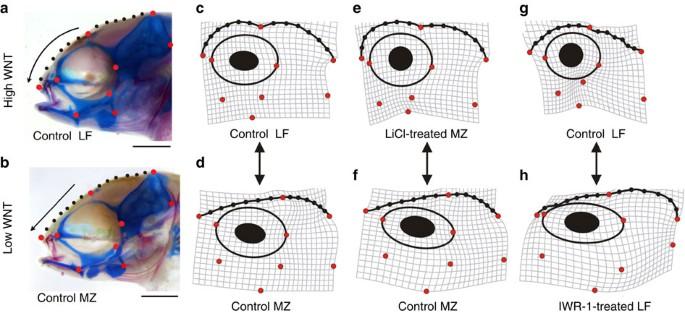Figure 4: Experimental manipulation of Wnt signalling recapitulates natural variation in craniofacial profile. LF larvae have endogenously higher levels of Wnt during preorbital (po) outgrowth compared to MZ. Skeletal preparations of the craniofacial skeleton are shown for LF (a) and MZ (b). Scale bars, 500μm. Deformation grids made in relation to a discriminant function analysis (DFA) reveal that much of the difference between LF (c) and MZ (d) control larvae with respect to craniofacial geometry relates to the slope of the craniofacial profile, which is steep in LF and shallow in MZ. Treatment of MZ larvae with the Wnt agonist, LiCl, results in a pronounced steepening of the profile of the po region of the skull (e) relative to control MZ (f) as revealed by DFA. Alternately, compared with control LF (g) experimental inhibition of Wnt signalling in LF larvae with the compound, IWR-1, results in the development of a significantly less steep and more shallow profile (h) as revealed by DFA. DFA results are depicted for each experiment comparing the craniofacial skeleton between animals with putatively higher (top row) versus lower (bottom row) levels of Wnt signalling during po development. All deformation grids are magnified × 3 to better visualize shifts in craniofacial geometry. Figure 4: Experimental manipulation of Wnt signalling recapitulates natural variation in craniofacial profile. LF larvae have endogenously higher levels of Wnt during preorbital (po) outgrowth compared to MZ. Skeletal preparations of the craniofacial skeleton are shown for LF ( a ) and MZ ( b ). Scale bars, 500μm. Deformation grids made in relation to a discriminant function analysis (DFA) reveal that much of the difference between LF ( c ) and MZ ( d ) control larvae with respect to craniofacial geometry relates to the slope of the craniofacial profile, which is steep in LF and shallow in MZ. Treatment of MZ larvae with the Wnt agonist, LiCl, results in a pronounced steepening of the profile of the po region of the skull ( e ) relative to control MZ ( f ) as revealed by DFA. Alternately, compared with control LF ( g ) experimental inhibition of Wnt signalling in LF larvae with the compound, IWR-1, results in the development of a significantly less steep and more shallow profile ( h ) as revealed by DFA. DFA results are depicted for each experiment comparing the craniofacial skeleton between animals with putatively higher (top row) versus lower (bottom row) levels of Wnt signalling during po development. All deformation grids are magnified × 3 to better visualize shifts in craniofacial geometry. Full size image We next set out to assess the degree to which the ancestral condition (that is, shallow craniofacial profile) could be recovered in the derived species by experimentally reducing levels of Wnt during preorbital outgrowth. To accomplish this we treated stage 17 LF larvae with 10–12 μM of the Wnt antagonist IWR-1. Consistent with our prediction, treated LF larvae developed a shallow craniofacial profile that was statistically similar to that of stage-matched MZ larvae ( Fig. 4g,h ). In all, these data strongly suggest that the evolution of a phenotypically derived, steeply descending profile in LF occurred, at least in part, via enhanced Wnt signalling during preorbital outgrowth. Expanded Wnt signalling leads to early and robust ossification While the specific molecular and cellular mechanisms through which Wnt signalling operates in the preorbital region of the skull requires further investigation, it possibly acts through osteoblast differentiation [12] . Evidence in support of this hypothesis includes the observation that LF exhibits early and robust mineralization of skeletal elements relative to MZ ( Fig. 5 ). Bones within the preorbital region of the teleost skull include those that comprise the upper jaw (for example, premaxilla and maxilla) as well as the anterior-most region of the skull, which supports the upper jaws as they open and close (for example, vomerine process) [8] . Soon after the initiation of preorbital outgrowth (that is, stage 22), LF and MZ differ with respect to the extent of mineralization of the premaxilla and maxilla (black arrows, Fig. 5 ). Mineralization of the anterior skull, including the vomerine process, also begins in LF well before MZ (white arrowheads, Fig. 5 ). In addition, the Wnt pathway member, lef1 , is discretely expressed within the preorbital region of the skull as bones in this area begin to form ( Supplementary Fig. 2 ). Specifically, at stage 18, the spatial expression domain of lef1 overlaps with that of the osteoblast marker, col1a1, in the developing skull (for example, parasphenoid) and upper jaws (for example, maxilla and premaxilla) ( Supplementary Fig. 2 ). Thus, the Wnt pathway is expressed within a discrete region of the skull where cichlids undergo differential rates/levels of mineralization. 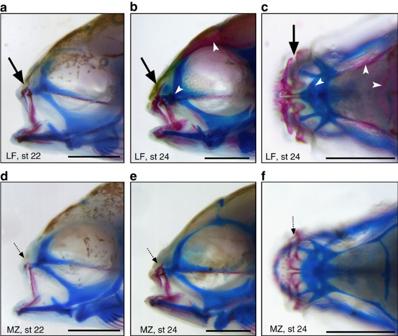Figure 5: The morphologically derived species with elevated Wnt signalling exhibits accelerated bone development. The craniofacial skeletons of LF (a–c) and MZ (d–f) are depicted from stages 22–24. Lateral views are depicted in (a,b) and (d,e). Dorsal views are shown in (c,f). The initial deposition of bone in the preorbital region of the skull (that is, upper jaw elements) is more intense in LF (a, large arrow) compared with MZ (d, dotted arrow). By stage 24, not only are the upper jaw elements more robustly mineralized in LF (b,c; large arrow) compared with MZ (e,f; dotted arrow), but LF have mineralized several more elements within the anterior region of the skull (b,c) compared with MZ (e,f), including the vomerine process (b,c; white arrowheads) and the margins of the prefrontal bone (b,c; black arrowheads). Scale bars, 500 μm. Figure 5: The morphologically derived species with elevated Wnt signalling exhibits accelerated bone development. The craniofacial skeletons of LF ( a – c ) and MZ ( d – f ) are depicted from stages 22–24. Lateral views are depicted in ( a , b ) and ( d , e ). Dorsal views are shown in ( c , f ). The initial deposition of bone in the preorbital region of the skull (that is, upper jaw elements) is more intense in LF ( a , large arrow) compared with MZ ( d , dotted arrow). By stage 24, not only are the upper jaw elements more robustly mineralized in LF ( b , c ; large arrow) compared with MZ ( e , f ; dotted arrow), but LF have mineralized several more elements within the anterior region of the skull ( b , c ) compared with MZ ( e , f ), including the vomerine process ( b , c ; white arrowheads) and the margins of the prefrontal bone ( b , c ; black arrowheads). Scale bars, 500 μm. Full size image In order to assess whether artificial expansion of Wnt signalling is sufficient to initiate bone development, we treated zebrafish with LiCl during a critical stage of preorbital development. Specifically, we treated zebrafish larvae with 10 mM of LiCl between 72–84 h ( n ~300 fish). Three phenotypic categories were noted with respect to craniofacial and bone development. The first, and most prevalent, phenotypic class (~75%) involved the variable loss of craniofacial bones and cartilages. Contrary to this loss-of-function phenotype, we also noted two distinct gain-of-function phenotypes in ~25% of treated animals. The first involved the development of ectopic bony nodules distributed across much of the body and fins ( Fig. 6a–c ). For example, pockets of mineralization were observed at regular intervals along the flank of the body ( Fig. 6b ), which occurred at the approximate location of the posterior lateral line placodes [14] . In addition, ectopic mineralization was variably observed within the fins, eyes and around the oral jaws ( Fig. 6c ). Pockets of ectopic mineralization along the top of the head also colocalized at high frequency with pigment cells. The observation of ectopic bone formation within tissues of putative neural crest and placode origins suggest that certain embryonic cell populations may be more responsive to Wnt levels with respect to bone formation. It is especially notable that areas of ectopic ossification correspond with areas of expanded Wnt signalling due to LiCl treatment, as seen in the Wnt reporter line, including within the pectoral fins (pf) and along the top of the skull ( Fig. 3c ). The second class of gain-of-function phenotype observed upon LiCl treatment was accelerated endogenous bone development. Compared with untreated control siblings ( Fig. 6d–f ), a subset of animals treated with 10 mM LiCl between 72–84 h ( Fig. 6g–i ) exhibited more extensive mineralization in various elements in the head, including the opercle, notochord and pharyngeal jaws. In general terms, both the loss- and gain-of-function phenotypes observed in larvae treated with LiCl suggest that variation in Wnt levels can have a potent effect on craniofacial development. More specific to our prediction, we demonstrate that elevated Wnt signalling is sufficient to drive bone development, and offer a putative mechanism through which Wnt is acting to influence variation in cichlid craniofacial development. 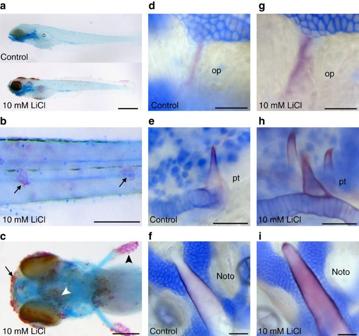Figure 6: Experimental upregulation of Wnt signalling leads to ectopic and accelerated bone development. (a) Zebrafish treated with 10 mM of LiCl between 3 and 3.5 dpf exhibit variable but striking gain-of-function phenotypes with respect to bone deposition. Scale bar, 500 μm. (b,c). Two general phenotypic categories were recognized—ectopic bone formation and accelerated development of endogenous bone. Fish were observed with ectopic bony nodules distributed across the body. Pockets of mineralization were observed at regular intervals down the body (b, arrows). Ectopic mineralization was also observed in the fins (c, black arrowhead), around the developing jaws (c, black arrow) and coincident with pigment cells on the roof of the skull (c, white arrowhead). Scale bars, 200 μm inb,c. Notably, these areas of ectopic bone formation generally correspond with regions in which Wnt signalling was observed in zebrafish. In addition, relative to control larvae (d,f), zebrafish treated with LiCl (g–i) exhibited accelerated development of endogenous mineralized tissue, including the opercle (op), pharyngeal teeth (pt) and the notochord (noto). Scale bars, 100 μm (d–i). Figure 6: Experimental upregulation of Wnt signalling leads to ectopic and accelerated bone development. ( a ) Zebrafish treated with 10 mM of LiCl between 3 and 3.5 dpf exhibit variable but striking gain-of-function phenotypes with respect to bone deposition. Scale bar, 500 μm. ( b , c ). Two general phenotypic categories were recognized—ectopic bone formation and accelerated development of endogenous bone. Fish were observed with ectopic bony nodules distributed across the body. Pockets of mineralization were observed at regular intervals down the body ( b , arrows). Ectopic mineralization was also observed in the fins ( c , black arrowhead), around the developing jaws ( c , black arrow) and coincident with pigment cells on the roof of the skull ( c , white arrowhead). Scale bars, 200 μm in b , c . Notably, these areas of ectopic bone formation generally correspond with regions in which Wnt signalling was observed in zebrafish. In addition, relative to control larvae ( d , f ), zebrafish treated with LiCl ( g – i ) exhibited accelerated development of endogenous mineralized tissue, including the opercle (op), pharyngeal teeth (pt) and the notochord (noto). Scale bars, 100 μm ( d – i ). Full size image The extreme phenotype exhibits environmental canalization We demonstrate above that expanded Wnt signalling is associated with limited preorbital outgrowth in LF, which in turn contributes to the development of a phenotypically derived craniofacial phenotype among Malawi cichlids. Since ecological specialization is predicted to result in a reduction in phenotypic plasticity [6] , we set out to test the hypothesis that the LF craniofacial skeleton is more robust to alternate feeding treatments (that is, environmentally canalized) than more generalized species. Here we focus on a comparison between two benthic foraging species LF and Tropheops ‘red cheek’ (TRC). This species of Malawi cichlid occupies a similar ecological niche as LF and possesses an adult craniofacial shape that is quantitatively more similar to LF than most other species in the lake [7] . However, as larvae TRC possess a relatively more elongate craniofacial profile that is similar to the more generalized species, MZ ( Supplementary Fig. 4a ). TRC therefore converge on an LF-like phenotype through later ontogenetic processes TRC also show allelic similarity to MZ at the β-catenin locus (that is, they carry the MZ allele), and are similarly tolerant to LiCl treatment as MZ (that is, develop the lock jaw phenotype at relatively higher concentrations of LiCl, Supplementary Fig. 4b ). Our plasticity experiment was intended to induce changes in jaw length by forcing animals to feed with either a biting or sucking mode of feeding (see Methods). Our data strongly support our hypothesis that LF possess a more environmentally canalized craniofacial skeleton. Whereas craniofacial architecture in LF was relatively invariant to diet treatment (average PD between diet treatment groups=0.0273), TRC showed a relatively stronger response to diet (average PD between diets=0.0406). We also performed a principal component analysis on treated fish. In LF, benthic- and limnetic-treated fish did not segregate along the primary axis of variation (PC1, t =0.16, df=35, P =0.8723), and shape variation along this axis was characterized by subtle shifts in premaxilla length and head depth (vector displacement of craniofacial landmarks, Fig. 7a ). Alternatively, TRC animals did segregate according to diet along PC1 ( t =5.89, df=37, P <0.0001), and exhibited larger shifts in head depth and craniofacial profile, which was steep in benthic animals and relatively shallow in animals forced to feed from the water column ( Fig. 7b ). These trends are highly consistent with those in the wild, where benthic and limnetic ecotypes are characterized by differences in preorbital length and profile—short and steeply descending in benthic forms, long and shallow slope in limnetic forms [7] , [8] . Thus, extreme ecological specialization in LF may have come at the expense of craniofacial variability. Below we offer a model connecting these two features of the skull in LF. 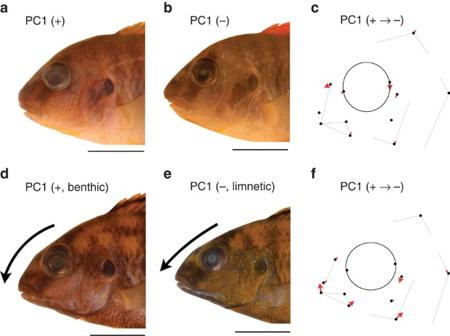Figure 7: The phenotypically derived species is more robust to environmental change. Families of LF and TRC were split and reared on distinct diet treatments to mimic benthic and limnetic modes of feeding. (a–c) Along the major axis of variation (PC1) the derived species, LF, shows no difference in craniofacial form when grouped by feeding treatment (t=0.16,n=35,P=0.8723). (a) Depicts an animal at the extreme positive end of PC1. (b) Shows an animal at the extreme negative end of PC1. (c) Illustrates the shape change associated variation along this axis as vector displacements at each craniofacial landmark. We consider this species to be more environmentally canalized. (d–f) Alternatively, in the more intermediate species, TRC, benthic and limnetic fish exhibited a marked shift in craniofaical form along this axis (t=5.89,n=37,P<0.0001). Animals from the benthic treatment developed, on average, more steeply descending craniofacial profiles (that is, positive PC1 scores) (d), whereas those from the limnetic treatment possessed more isognathus jaws (that is, negative PC1 scores) (e). These plastic differences are highly similar to evolved differences among benthic and limnetic species in the wild, including craniofacial profile (black arrows;d,e), as well as a more streamlined head and up turned jaw (vector displacement of craniofacial landmarks,f). Scale bars, 1 cm. Figure 7: The phenotypically derived species is more robust to environmental change. Families of LF and TRC were split and reared on distinct diet treatments to mimic benthic and limnetic modes of feeding. ( a – c ) Along the major axis of variation (PC1) the derived species, LF, shows no difference in craniofacial form when grouped by feeding treatment ( t =0.16, n =35, P =0.8723). ( a ) Depicts an animal at the extreme positive end of PC1. ( b ) Shows an animal at the extreme negative end of PC1. ( c ) Illustrates the shape change associated variation along this axis as vector displacements at each craniofacial landmark. We consider this species to be more environmentally canalized. ( d – f ) Alternatively, in the more intermediate species, TRC, benthic and limnetic fish exhibited a marked shift in craniofaical form along this axis ( t =5.89, n =37, P <0.0001). Animals from the benthic treatment developed, on average, more steeply descending craniofacial profiles (that is, positive PC1 scores) ( d ), whereas those from the limnetic treatment possessed more isognathus jaws (that is, negative PC1 scores) ( e ). These plastic differences are highly similar to evolved differences among benthic and limnetic species in the wild, including craniofacial profile (black arrows; d , e ), as well as a more streamlined head and up turned jaw (vector displacement of craniofacial landmarks, f ). Scale bars, 1 cm. Full size image Wnt signalling has been implicated in mediating craniofacial [9] and bone [11] development. With respect to craniofacial development, most work has focused on roles for Wnts in mediating relatively early stages of neural crest cell development (for example, induction, migration, and so on) [9] , [10] . Here we examine slightly later events in development—outgrowth of the preorbital region of the skull—in both cichlids and zebrafish. In terms of both expression and functional manipulation of the Wnt pathway, we observed markedly similar affects. In both species, Wnt signalling components are expressed in a discrete domain along the anterior portion of the developing skull. Furthermore, expanded Wnt signalling via chemical modulation in both cichlids and zebrafish larvae during periods of normal preorbital outgrowth severely attenuates this region of the skull. Cichlids and zebrafish represent distinct orders of bony fish separated by ~300 million years of evolution [15] , and yet these data support the idea that they possess a similar mode of skull outgrowth, at least in terms of Wnt signalling. These data are especially notable with respect to patterns of diversification among various fish lineages. Modulation of the size of the preorbital region of the skull has figured prominently in the adaptive radiation of sunfishes (Centrarchidae) [16] , wrasses (Labridae) [17] , damselfish (Pomacentridae) [18] , stickleback (Gasterosteidae) [19] , charr/whitefish (Salmonidae) [6] , [20] and cichlids (Cichlidae) [7] , [8] , [21] . Our data raise the interesting possibility that a conserved molecular mechanism may underlie these independent evolutionary radiations. At the very least, they offer a candidate pathway for future investigations in lineages that are less experimentally tractable but show similar patterns of divergence. All cichlid larvae possess a steeply rounded preorbital profile at early stages of craniofacial development ( Fig. 8a ). In most species, outgrowth of this region of the skull commences during larval stages and continues into adult stages of development. In the phenotypically derived species, LF, preorbital outgrowth is severely attenuated during larval stages. We therefore consider this novel phenotype to be an example of a paedomorphism. The adaptive value of a steeply descending craniofacial profile with respect to foraging efficiency has been examined and discussed previously, and includes an increased ability of the craniofacial skeleton to mitigate strain due to a highly specialized biting mode of feeding [8] . 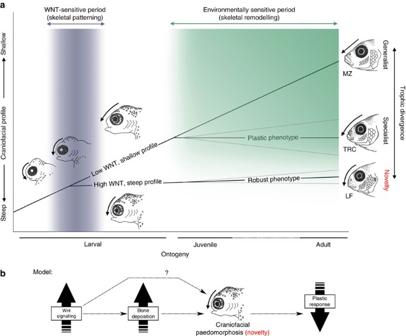Figure 8: Expanded Wnt-signalling is associated with the evolution of phenotypic novelty and reduced craniofacial variability in Lake Malawi cichlids. Our model is depicted as a schematic graph (a) and a flow-chart (b). All early cichlid larvae possess conspicuously rounded craniofacial profiles. Beginning at larval stages, outgrowth of the preorbital (po) region of the skull results in the profile becoming progressively less rounded. Discrete Wnt expression within the po region of the larval head suggests that this pathway is associated with the development of this anatomical unit. Expanded Wnt signalling is associated with the retention of a rounded profile throughout ontogeny (paedomorphosis), and the evolution of a craniofacial architecture that is unique to all other East African cichlids7. Experimental manipulation of the Wnt pathway during this sensitive period can recapitulate both generalist and novel phenotypes. We suggest that expanded Wnt signalling acts to lock into place an early larval phenotype, possibly via accelerated bone development. This mechanistic hypothesis is supported by experiments in zebrafish that show that LiCl treatment results in expanded Wnt signalling, ectopic bone development and accelerated development of endogenous craniofacial bones. Finally, we show that this novel, paedomorphic phenotype is more robust to environmental input, decreasing craniofacial variability within this lineage. In all, our data suggest that the evolution of craniofacial novelty has come at the expense of variability, which may ultimately limit evolutionary potential. Figure 8: Expanded Wnt-signalling is associated with the evolution of phenotypic novelty and reduced craniofacial variability in Lake Malawi cichlids. Our model is depicted as a schematic graph ( a ) and a flow-chart ( b ). All early cichlid larvae possess conspicuously rounded craniofacial profiles. Beginning at larval stages, outgrowth of the preorbital (po) region of the skull results in the profile becoming progressively less rounded. Discrete Wnt expression within the po region of the larval head suggests that this pathway is associated with the development of this anatomical unit. Expanded Wnt signalling is associated with the retention of a rounded profile throughout ontogeny (paedomorphosis), and the evolution of a craniofacial architecture that is unique to all other East African cichlids [7] . Experimental manipulation of the Wnt pathway during this sensitive period can recapitulate both generalist and novel phenotypes. We suggest that expanded Wnt signalling acts to lock into place an early larval phenotype, possibly via accelerated bone development. This mechanistic hypothesis is supported by experiments in zebrafish that show that LiCl treatment results in expanded Wnt signalling, ectopic bone development and accelerated development of endogenous craniofacial bones. Finally, we show that this novel, paedomorphic phenotype is more robust to environmental input, decreasing craniofacial variability within this lineage. In all, our data suggest that the evolution of craniofacial novelty has come at the expense of variability, which may ultimately limit evolutionary potential. Full size image Notably, limited preorbital outgrowth in LF is associated with accelerated craniofacial bone development. Whether these two events are molecularly linked or developmentally coincident remains to be investigated ( Fig. 8b ). However, given (1) experimental manipulation of the Wnt pathway recapitulates natural variation in preorbital profile, (2) experimental elevation of Wnt signalling is sufficient to drive bone development, and (3) known roles for Wnt signalling in mediating bone development in other vertebrates [12] , we offer the hypothesis that the evolution of craniofacial novelty in Lake Malawi cichlids is due, at least in part, to selection for accelerating bone development and a steep craniofacial profile via expanded Wnt signalling. While LF showed little response with respect to craniofacial profile when fed alternate diets, the primary axis of variation between benthic/limnetic TRC involved discrete changes in both head depth and preorbital profile. It is noteworthy that this plastic response was broadly similar to the effects of LiCl/IWR-1 treatments in larvae, and it is possible that a plastic response to a benthic diet later in ontogeny also involves an upregulation of the Wnt pathway. A benthic foraging strategy is likely to involve a higher degree of mechanical stress on craniofacial bones (that is, biting versus suction feeding), which should in turn result in the reinforcement of these bones through the process of remodelling (for example, Wolff’s law [22] ). A direct link between mechanical stress, bone remodelling and Wnt signalling is well established in the literature [23] , wherein increased mechanical stress levels are associated with an upregulation of β -catenin/Wnt signalling and subsequently higher levels of mineralization. These considerations raise the interesting possibility that the extreme craniofacial phenotype possessed by LF evolved through a process of genetic assimilation through changes in the Wnt pathway. Waddington [24] coined the term canalization to describe the property of developmental systems to produce the same phenotype regardless of the conditions under which development occurs. Without knowing the underlying mechanisms, he posited an epigenetic landscape metaphor wherein development could be visualized much like a marble (that is, metaphor for an embryo) rolling down to the lowest point of elevation. The wider the valley through which the marble rolls, the greater the expected variation in development. Waddington suggested that natural selection could increase or decrease variation in developmental systems by widening or narrowing the valleys on the landscape. Since natural selection targets phenotypic variation [25] , the evolution of canalized phenotypes (for example, narrowed valleys) could limit future evolutionary potential (that is, evolvablity). Relative to other East-African cichlids, LF is pushing the limits of craniofacial diversity, as it defines the extreme outer edge of phenotypic variation in craniofacial shape [7] . Both our expression analyses and small molecule data suggest that this is due, at least in part, to expanded Wnt signalling, which serves to ‘lock’ an adult phenotype into place early in ontogeny. While this novel developmental trajectory has resulted in the evolution of phenotypic novelty and increased ecological success, it is also associated with the evolution of environmental canalization and decreased variability ( Fig. 8 ). In other words, LF is less able to remodel its feeding apparatus over ontogeny in response to changes in foraging habitat. This putative tradeoff may explain both the biogeography and evolutionary history of this lineage. Specifically, the lake-wide distribution of LF may have been facilitated by its unique and environmentally canalized trophic apparatus, but the Labeotropheus genus is also one of the most species-poor lineages in the lake with only two species within the genus. While fewer species does not necessarily translate to a reduced ability to evolve, it is consistent with the hypothesis that ecological specialization has come at the expense of variability and evolutionary potential. An important caveat to our approach is that Wnt signalling is not being manipulated in a tissue-specific manner. Thus, cell-autonomous effects are difficult to discern from secondary effects on phenotype. To mitigate this potentially confounding issue our small-molecule treatments were targeted to narrow periods of embryonic development (for example, preorbital outgrowth and bone development), which will limit potentially broader effects on anatomy. In addition to the ability to manipulate pathways in a time-specific manner, a small-molecule approach offers other advantages. For one, it enables the dosing and high-throughput analysis of many hundreds of animals, thus allowing for a rigorous statistical assessment of subtle effects on morphology. It also offers the ability to alter the expression of pathways in a continuous, dose-specific fashion rather than completely knocking out their function. This allows for the phenotypic effects of a response to be related to concentration (that is level of expression), which is very relevant for evolutionary systems that exhibit a gradient of phenotypic variation. We take advantage of each of these attributes here. Nevertheless, the primary cellular behaviours that underlie the phenotypes described above will require further investigation. Our results offer a potential molecular inroad to gain a better and more mechanistic understanding of canalization and the ways in which variation can be shaped by development and respond to selection. In particular, we find that Wnt signalling is linked to both variation and variability in cichlid craniofacial form. Expanded levels of Wnt are associated with the evolution of a derived morphology by locking into place an early larval phenotype, and this process is associated with an increase in environmental canalization as well as increased sensitivity to molecular perturbation. In both cases, this should translate into the production of a phenotype well suited for its current niche, but less able to adapt (both in the short and long terms) to changes in its environment. Maintenance of fish species All fish used in this study were bred, reared and killed according to protocols approved by the Institutional Animal Care and Use Committee (IACUC) at the University of Massachusetts. Cichlid species were collected from Lake Malawi, and reared in 40-gallon glass aquaria, at 28.5 °C±1°C on a 14 h light/10 h dark cycle. All larvae were F 1 - or F 2 -derived from wild-caught stock, and obtained by natural matings. Lake Malawi cichlid females mouth brood their young, and brooding females are easily identified by an enlarged buccal cavity. We generally extracted embryos from mouthbrooding females between 3–4dpf (stages 10–14). Embryos were incubated in 1-l glass beakers with ~900 ml of system water plus 2–3 drops of methylene blue, and kept at 28.5 °C±1 °C. An aeration stone was placed at the bottom of the flask to provide enough air to keep the embryos vigorously swirling at the bottom of the flask. Embryo medium was changed every 2 days. Cichlid staging was according to the study by Fujimura et al. [26] Wild-type (EKW) and transgenic (Tg(7xTCF-Xla.Siam:GFP) [27] ) zebrafish ( Danio rerio ) were maintained and bred in a separate recirculating system from cichlids, but were likewise kept at 28.5 °C±1 °C in a 14 h light/ 10 h dark cycle. Embryos were collected by natural matings and staged according to Kimmel et al. [28] In situ hybridization Embryos were fixed in 4% paraformaldehyde and stored in 100% methanol for WISH. Digoxigenin-labelled RNA probe design and WISH analyses were performed using standard methods [29] . Probes were generated from cDNA sequence derived from partial genome assemblies of several Lake Malawi cichlids [11] . Multiple specimens (3–5) were used for each probe, and WISH was repeated at least once for every probe and species to control for variation across experiments. Small-molecule manipulation of Wnt-signalling We first observed and compared the ontogeny of early jaw development in LF and MZ. We identified a notable period of preorbital outgrowth between 6–8 dpf (stages 17–21) that resulted in differences in preorbital length between species. Following this we designed an experiment that would alter the expression of the Wnt pathway before morphological changes in jaw length. We hypothesized that a range of concentrations of LiCl, an activator of the Wnt pathway, would provide a means to investigate the role of this pathway in determining preorbital length. Single broods of early stage 17 (5.5 dpf) embryos were divided and either dosed for a period of 6 h across a range of concentrations of LiCl (starting at 0.5 mM, increasing to 1 mM and increasing further in increments of 1 mM to a maximum concentration of 8 mM) or kept in system water (control). Following treatment larvae were washed in system water three times, and placed back into a clean beaker to be reared to stage 21 (8 dpf). At this stage embryos were killed using MS-222 and fixed in 4% paraformaldehyde overnight before acid-free clearing and staining of skeletal elements [30] . For all experimental concentrations of LiCl, two to three families of either LF or MZ were used. Total sample sizes ranged from 20–42 individuals for each species at every concentration. Including controls, a total of 494 larvae were examined ( n =264 MZ, n =230 LF). TRC are aggressive and relatively more difficult to breed in the lab. Access to embryos from these animals was therefore more limited. A total of 42 TRC larvae were treated across a range of LiCl concentrations (that is, 0, 3, 4, 6 and 8 mM), with 8–9 individuals per treatment. These animals were used to assess the frequency of developing a lock jaw phenotype in response to LiCl treatment. Our LiCl experiments were broad and robust, and intended to assess the extent to which various species respond to various concentrations of this compound with respect to craniofacial development. Performing a similarly broad experiment using a Wnt antagonist is outside the scope of this study, in terms of both time and expense. Nevertheless, based on the results of the LiCl experiment, we wanted to see whether knockdown of Wnt signalling would result in a predictable response. Specifically, given that upregulation of the Wnt pathway resulted in the development of a steep craniofacial profile, we predicted that downregulation would result in the development of a more shallow craniofacial profile. In order to test this prediction, we treated stage 17 LF larvae with the Wnt antagonist [13] IWR-1 (Enzo Life Sciences) for 12 h. Control animals were incubated in DMSO. Larvae were treated with 10–12 μM of IWR-1, based on previously published data in cichlids [31] , [32] . Following treatment larvae were washed in system water three times, and placed back into a clean beaker to be reared to stage 21 (8 dpf), when they were cleared and stained as above. In order to assess the degree to which the effects of LiCl treatment on craniofacial development are evolutionary conserved, we treated 48 h zebrafish with 10mM of LiCl for 6 h ( n =54, mixed families). Larva were cleared and stained at 5 dpf as above and assessed for craniofacial defects relative to control larvae ( n =31). In order to assess the extent to which LiCl treatment affected bone development 72 h zebrafish were treated with 10 mM of LiCl for 12 h ( n =298, mixed families), cleared and stained at 5 dpf, and compared to control larvae ( n =87). Morphometrics A quantitative geometric morphometric analysis of shape change in response to experimental treatments of LiCl was conducted for all of the embryos. This analysis covered shape variation from the entire craniofacial region, but with a focus on the profile of the dorsal region extending from the occipital crest to the maxillae. Following clearing and staining all embryos were photographed using a Leica DFC450 camera mounted to Leica MF15 stereomicroscope. All photos, which included a scale factor, were taken on the left lateral view of the embryos that were positioned in 80% glycerol. Landmarks and semilandmarks were collected from photos using the software TPSDig2 (ref. 33 ). Semilandmarks were initially collected as two curves on the dorsal region, with data being reduced to six landmarks per curve using the software semithinner [34] . Regular landmarks and semilandmarks were then defined using the software TPSutil [33] , and raw data for statistical analysis was obtained by sliding semilandmarks using the chord distance function in TPSrelw [33] . Raw data were provided in two forms, consisting of landmark coordinates for each individual that were corrected for variation in size, rotation and in the form of partial warp scores, which quantified the change in shape a reference configuration of landmarks would require to become an individual. Statistics We aimed to determine the effects that altered Wnt activity could have on craniofacial shape, and whether this impacted LF and MZ differently. Therefore, we modelled the potential effects of LiCl concentration and species on multivariate shape using a mulitavariate analysis of variance (MANOVA) in all 494 animals. For this MANOVA we used partial warp scores as our raw data, and included concentration, species and their interaction as factors using base functions in the R statistical language [35] . We used PD in order to assess the degree of deviation (that is, ‘distance’) of craniofacial shape in response to LiCl treatment from a reference configuration. Specifically, we calculated the PD of every individual from a reference configuration derived from the average shape of the control MZ. We then plotted the mean and 95% confidence interval of PDs for each concentration and species. Confidence intervals were calculated using the pastecs package in R, and plots were created using the plotrix package in R [35] . To examine natural variation, and the effect of our experiments that enhanced or inhibited Wnt signalling we employed a series of linear discriminant function analyses using the MASS package in R [35] . This included comparisons between control LF and MZ, control MZ and those treated with 7–8 mM of LiCl, and control LF and those treated with 10–12 μM of IWR-1. The shape changes associated with our experimental treatments and natural differences were visualized by regressing shape data against canonical root scores obtained from their respective discriminant function analys model using TPSregr [33] . To get a sense of differences in a common morphospace all pairwise PDs between these groups were calculated using the software Coordgen [34] . Developmental plasticity LF is a phenotypically derived species that ‘locks’ its adult phenotype into place early in development, due, at least in part, to expanded Wnt signalling. TRC is a close ecological competitor of LF [36] , and as an adult possesses a craniofacial skeleton that is similar to LF, but it’s larval form is more similar to that of MZ, a more generalized species. We therefore hypothesized that the craniofacial skeleton of LF would be robust to environmental inputs, relative to TRC. To test this, we split families of LF and TRC and reared them on identical diets, but under distinct kinematic conditions—‘benthic’ and ‘limnetic’. For the benthic treatment, we ground a mixture of high-quality algae flake food, algae wafers and freeze-dried daphnia. We then embedded this mixture in 1.5% food-grade agar (Carolina Biological Supply Co., Burlington, NC, USA) and spread it over store-bought lava rocks. These ‘algae rocks’ were allowed to air dry overnight and then sunk to the bottom of aquaria. This treatment was intended to induce a ‘scraping’ mode of feeding that is typical of many rock-dwelling cichlid species in the wild, including LF and TRC. For the alternate ‘limnetic’ treatment, the same ground food mixture was simply sprinkled into aquaria. In addition, two to three times a week, limnetic animals were given live daphnia. Foraging treatments began at 2 months of age when animals were big enough to be housed in 40-gallon aquaria. Up until this point all animals were fed a typical larval diet of ground flake food. Feeding treatments were performed for 5 months, at which point animals were killed, fixed in 4% PFA and stored in 75% ethanol. In total 35 LF (split approximately equally between treatments) and 37 TRC (again, split roughly equally) were analysed. Animals were dissected to reveal functionally salient landmarks, photographed in the left lateral view using a Canon EOS digital camera (Canon EOS Rebel, Lake Success, NY, USA) and digital landmarks were placed on their heads using TPSdig [33] and according to Cooper et al. [7] The extent to which feeding treatments affected craniofacial shape was assessed using PDs (as above) and relative warps analysis following Cooper et al. [7] How to cite this article: Parsons, K. J. et al. Wnt signalling underlies the evolution of new phenotypes and craniofacial variability in Lake Malawi cichlids. Nat. Commun. 5:3629 doi: 10.1038/ncomms4629 (2014).